PI(4,5)P2 5-phosphatase A regulates PI3K/Akt signalling and has a tumour suppressive role in human melanoma Inositol polyphosphate 5-phosphatases can terminate downstream signalling of phosphatidylinositol-3 kinase; however, their biological role in the pathogenesis of cancer is controversial. Here we report that the inositol polyphosphate 5-phosphatase, phosphatidylinositol 4,5-bisphosphate 5-phosphatase, has a tumour suppressive role in melanoma. Although it is commonly downregulated in melanoma, overexpression of phosphatidylinositol 4,5-bisphosphate 5-phosphatase blocks Akt activation, inhibits proliferation and undermines survival of melanoma cells in vitro , and retards melanoma growth in a xenograft model. In contrast, knockdown of phosphatidylinositol 4,5-bisphosphate 5-phosphatase results in increased proliferation and anchorage-independent growth of melanocytes. Although DNA copy number loss is responsible for downregulation of phosphatidylinositol 4,5-bisphosphate 5-phosphatase in a proportion of melanomas, histone hypoacetylation mediated by histone deacetylases HDAC2 and HDAC3 through binding to the transcription factor Sp1 at the PIB5PA gene promoter appears to be another commonly involved mechanism. Collectively, these results establish the tumour suppressive role of phosphatidylinositol 4,5-bisphosphate 5-phosphatase and reveal mechanisms involved in its downregulation in melanoma. Aberrant activation of survival-signalling pathways causes uncontrolled cell proliferation and resistance to apoptosis, and has an important role in cancer development, progression and resistance to treatment [1] , [2] . In melanoma, activation of the mitogen-activated protein kinase pathway stems primarily from activating mutations of BRAF [3] , [4] . Targeting mutant BRAF has achieved unprecedented responses in clinical trials in metastatic melanoma patients [5] , [6] , [7] . However, primary and acquired resistance, which is commonly associated with activation of other survival pathways, in particular the phosphatidylinositol-3 kinase (PI3K)/Akt pathway, remain a major obstacle in the quest for curative treatment [8] , [9] , [10] , [11] . Indeed, activation of PI3K/Akt signalling has been shown to cooperate with mutant BRAF in melanomagenesis using in vivo models [12] , [13] . PI3K signalling is initiated with the engagement of extracellular growth factors to receptor tyrosine kinases. This results in recruitment of PI3K to plasma membrane-anchored receptors where it is activated, leading to increases in the production of phosphatidylinositol(3,4) bisphosphate (PI(3,4)P 2 ) and phosphatidylinositol(3,4,5)trisphosphate (PI(3,4,5)P 3 ), which in turn bind to and activate multiple downstream effectors [14] , [15] , [16] . Among them is Akt, which is activated by two phosphorylation events at Thr308 and Ser473 involving phosphoinositide-dependent kinase-1 and phosphoinositide-dependent kinase-2, respectively [17] , [18] . Although phosphorylation at Thr308 partially activates Akt, its full activation requires phosphorylation at Ser473 (refs 17 , 18 , 19 , 20 ). Although both PI(3,4)P 2 and PI(3,4,5)P 3 are involved, many studies have suggested that PI(3,4,5)P 3 is more important for the activation of Akt [21] , [22] , [23] , [24] . The intracellular levels of PI(3,4,5)P 3 are negatively regulated through dephosphorylation by two classes of inositol polyphosphate phosphatases [23] , [25] . The 3-phosphatase, phosphate and tensin homologue deleted on chromosome 10 (PTEN) dephosphorylates the third position of PI(3,4,5)P 3 to generate PI(4,5)P 2 (refs 25 , 26 ), whereas inositol polyphosphate 5-phosphatases (5-phosphatases), such as Src homology 2-containing inositol 5-phosphatase (SHIP), SHIP2 and phosphatidylinositol 4,5-bisphosphate 5-phosphatase (PIB5PA)/proline-rich inositol polyphosphate phosphatase, dephosphorylate the fifth position to produce PI(3,4)P 2 (ref. 27 ). The latter is in turn subjected to dephosphorylation by inositol polyphosphate 4-phosphatase type I (INPP4A) and type II (INPP4B) at the fourth position to terminate PI3K signalling [28] , [29] , [30] . Although PTEN is a well-established tumour suppressor owing to its inhibitory effect on the PI3K/Akt pathway [25] , [26] , recently INPP4B also has been shown to inhibit PI3K signalling and to suppress malignant behaviour of breast and prostate cancer cells [28] , [29] , [30] . However, the inhibitory effect of 5-phosphatases on PI3K/Akt signalling remains controversial. This is in part because their product PI(3,4)P 2 is a positive regulator of Akt activation [31] , [32] . Nevertheless, SHIP inhibits Akt activation in hematopoietic cells and PIB5PA similarly inhibits PI3K signalling in neurites and chicken embryo fibroblasts [21] , [24] , [27] . Of interest, high levels of PIB5PA have been reported to correlate with limited tumour progression and better prognosis in breast cancer patients [33] . The PI3K/Akt pathway is constitutively activated in up to 70% of melanomas [4] , [34] . This is frequently associated with downregulation or loss of PTEN mediated by genetic or epigenetic mechanisms and, in some cases, is related to activating mutations in NRAS , PI3KCA (the gene encoding the p110α catalytic subunit of PI3K) and genes of receptor tyrosine kinases, such as c-KIT , in subsets of melanomas [4] , [35] , [36] . In this report, we provide evidence that the decreased expression of the 5-phosphatase PIB5PA also contributes to elevated activation of PI3K/Akt signalling, and that PIB5PA has a tumour suppressive role in melanoma. Moreover, we show that recruitment of histone deacetylase (HDAC)2 and HDAC3 through binding to Sp1 at the PIB5PA promoter has an important role in suppression of PIB5PA in melanoma cells. PIB5PA is downregulated in human melanoma We examined the expression of PIB5PA in relation to melanoma development and progression by use of immunohistochemistry in tissue microarrays (TMAs) constructed from 100 formalin-fixed paraffin-embedded melanocytic tumours ( Supplementary Table S1 ). The results revealed that the PIB5PA expression was frequently reduced or lost in melanomas compared with nevi ( Fig. 1a and Supplementary Fig. S1 ), although there was no significant difference in PIB5PA levels between thin and thick primary melanomas, or between primary and metastatic melanomas ( Fig. 1a and Supplementary Table S1 ). Of note, although there was no significant relationship between PIB5PA levels and activation of Akt as determined by the expression of pSer473-Akt, the decreased expression of PIB5PA was positively correlated with PTEN (that was also decreased or lost in melanomas; Fig. 1a and Supplementary Tables S1 and S2 ). In particular, approximately one-third (6/17) of PTEN-null melanomas also displayed PIB5PA deficiency ( Supplementary Fig. S1 ). These results suggest that downregulation of PIB5PA and PTEN may cooperate to contribute to hyperactivation of PI3K/Akt signalling in melanoma. In support, examination of 20 fresh metastatic melanoma isolates by western blotting also showed that PIB5PA levels were positively correlated with PTEN ( Fig. 1c ). Similar to the finding in TMAs, there was no overall correlation between PIB5PA and pSer473-Akt levels in fresh melanoma isolates ( Supplementary Fig. S2 ). Nevertheless, fresh isolates deficient in both PTEN and PIB5PA ( n =3) had higher levels of pSer473-Akt compared with those expressing at least one of the proteins ( n =17; Fig. 1e ). 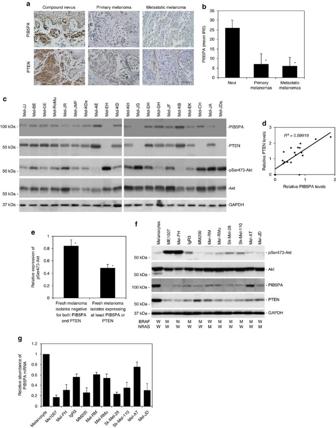Figure 1: PIB5PA is downregulated in melanoma cells. (a) Representative microphotographs of immunohistochemistry staining of PIB5PA and PTEN (brown) on melanocytic tumour tissue sections. Scale bar, 100 μm. (b) Quantification of PIB5PA expression levels in melanocytic tumours (see alsoSupplementary Tables S1 and S2, and Supplementary Fig. S1). Data shown are mean immunoreactive score (IRS)±s.e.m.; Student’st-test; *P<0.01. (c) Whole-cell lysates from fresh melanoma isolates were subjected to western blot analysis. Data shown are representative of three individual western blot analyses. (d) Representative regression analysis of relationship between PIB5PA and PTEN expression as shown inc. Levels of PIB5PA and PTEN were normalized to those of GAPDH. Quantification of each band was determined using NIH Image J. (e) Comparison of pSer473-Akt levels between fresh melanoma isolates negative for both PIB5PA and PTEN, and those expressing at least one of the proteins. Levels of pSer473-Akt were normalized to those of total Akt. Quantification of each band was determined using NIH Image J (n=3, mean±s.e.m.; Student’st-test; *P<0.05). (f) Whole-cell lysates from pooled melanocytes of three different lines (HEMa-LP, HEMa-DP and HEMn-LP) and melanoma cell were subjected to western blot analysis. Data shown are representative of three individual experiments. BRAF and NRAS mutational status of the cell lines was also indicated. W, wild-type; M, BRAFV600Eor NRASQ61Rmutation. (g) Quantitative reverse transcription–PCR analysis of total RNA extracted from melanocytes and melanoma cells showing that PIB5PA mRNA levels are commonly downregulated in melanoma cells compared with melanocytes. The relative abundance of PIB5PA mRNA expression in melanocytes was arbitrarily designated as 1 (n=3, mean±s.e.m.). Figure 1: PIB5PA is downregulated in melanoma cells. ( a ) Representative microphotographs of immunohistochemistry staining of PIB5PA and PTEN (brown) on melanocytic tumour tissue sections. Scale bar, 100 μm. ( b ) Quantification of PIB5PA expression levels in melanocytic tumours (see also Supplementary Tables S1 and S2 , and Supplementary Fig. S1). Data shown are mean immunoreactive score (IRS)±s.e.m. ; Student’s t -test; * P <0.01. ( c ) Whole-cell lysates from fresh melanoma isolates were subjected to western blot analysis. Data shown are representative of three individual western blot analyses. ( d ) Representative regression analysis of relationship between PIB5PA and PTEN expression as shown in c . Levels of PIB5PA and PTEN were normalized to those of GAPDH. Quantification of each band was determined using NIH Image J. ( e ) Comparison of pSer473-Akt levels between fresh melanoma isolates negative for both PIB5PA and PTEN, and those expressing at least one of the proteins. Levels of pSer473-Akt were normalized to those of total Akt. Quantification of each band was determined using NIH Image J ( n =3, mean±s.e.m. ; Student’s t -test; * P <0.05). ( f ) Whole-cell lysates from pooled melanocytes of three different lines (HEMa-LP, HEMa-DP and HEMn-LP) and melanoma cell were subjected to western blot analysis. Data shown are representative of three individual experiments. BRAF and NRAS mutational status of the cell lines was also indicated. W, wild-type; M, BRAF V600E or NRAS Q61R mutation. ( g ) Quantitative reverse transcription–PCR analysis of total RNA extracted from melanocytes and melanoma cells showing that PIB5PA mRNA levels are commonly downregulated in melanoma cells compared with melanocytes. The relative abundance of PIB5PA mRNA expression in melanocytes was arbitrarily designated as 1 ( n =3, mean±s.e.m.). Full size image We also examined the expression of PIB5PA in a panel of melanoma cell lines, which had varying status for the most common mutations in BRAF (BRAF V600E ) and NRAS (NRAS Q61R ), but harboured no mutations in other key components of the PI3K/Akt pathway, including PTEN , PI3KCA , EGFR and c-KIT ( Fig. 1f ). The melanoma cell lines commonly expressed lower levels of PIB5PA and PTEN than pooled melanocytes of three different lines (HEMa-LP, HEMa-DP and HEMn-LP; pooled normal melanocytes were used to simplify analysis, as these normal melanocyte lines expressed similarly higher levels of PIB5PA than melanoma cell lines; Fig. 1f and Supplementary Fig. S3 ). Although there was no correlation between the levels of pSer473-Akt and PIB5PA, the two lines (ME1007 and Mel-FH) expressing particularly low levels of PIB5PA and PTEN displayed the highest levels of pSer473-Akt ( Fig. 1f ). Collectively, these results indicate that PIB5PA is suppressed in melanoma cells, and suggest that low levels of PIB5PA may contribute to activation of the PI3K/Akt pathway. PIB5PA inhibits proliferation and survival in melanoma cells To investigate the effect of PIB5PA on PI3K/Akt signalling in melanoma cells, we introduced an haemagglutinin (HA)-tagged PIB5PA construct or a HA-tagged mutant PIB5PA construct (catalytically inactive PIB5PA SKICH ) into ME1007 and Mel-FH cells ( Fig. 2a and Supplementary Fig. S4 ). Overexpression of PIB5PA, but not the mutant, caused a decrease in pSer473-Akt in melanoma cells ( Fig. 2a and Supplementary Fig. S4 ). Although overexpression of PIB5PA triggered apoptosis in a proportion of ME1007 and Mel-FH cells ( Fig. 2b ), inhibition of cell proliferation appeared to be the predominant functional consequence as shown in 5-bromo-2′-deoxyuridine (BrdU) incorporation and clonogenic assays ( Fig. 2d ). In support of a role for inhibition of PI3K/Akt activation in these events, phosphorylation of the downstream targets, GSK3β and Bad, was decreased, whereas the expression of p27 and p21, two major negative regulators of cell cycle progression that can be inhibited directly or indirectly by Akt signalling [37] , was upregulated in both cell lines overexpressing PIB5PA ( Fig. 2a ). 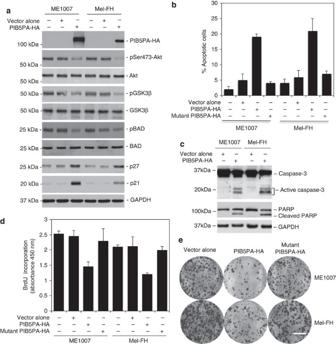Figure 2: Transient overexpression of PIB5PA inhibits cell proliferation and survival. (a) Whole-cell lysates from ME1007 and Mel-FH cells, either non-transfected or transfected with empty vector-HA or PIB5PA-HA constructs, were subjected to western blot analysis. Data shown are representative of three individual experiments. (b–e) ME1007 and Mel-FH cells were transiently transfected with empty HA, PIB5PA-HA, or mutant PIB5PA (PIB5PASKICH)-HA constructs. (b) Seventy-two hours later, apoptotic cells were quantitated by measurement of sub-G1 DNA content (n=3, mean±s.e.m.). (c) Forty-eight hours later, whole-cell lysates were subjected to western blot analysis. Data shown are representative of three individual experiments. (d) Seventy-two hours later, cells were subjected to proliferation assays using the BrdU incorporation method (n=3, mean±s.e.m.). (e) Twenty-four hours later, viable cells (2,000 cells per well in six-well plates) were allowed to grow for 12 days before being fixed with methanol and stained with crystal violet. Data shown are representative of three individual experiments. Scale bar, 1 cm. Figure 2: Transient overexpression of PIB5PA inhibits cell proliferation and survival. ( a ) Whole-cell lysates from ME1007 and Mel-FH cells, either non-transfected or transfected with empty vector-HA or PIB5PA-HA constructs, were subjected to western blot analysis. Data shown are representative of three individual experiments. ( b – e ) ME1007 and Mel-FH cells were transiently transfected with empty HA, PIB5PA-HA, or mutant PIB5PA (PIB5PA SKICH )-HA constructs. ( b ) Seventy-two hours later, apoptotic cells were quantitated by measurement of sub-G1 DNA content ( n =3, mean±s.e.m.). ( c ) Forty-eight hours later, whole-cell lysates were subjected to western blot analysis. Data shown are representative of three individual experiments. ( d ) Seventy-two hours later, cells were subjected to proliferation assays using the BrdU incorporation method ( n =3, mean±s.e.m.). ( e ) Twenty-four hours later, viable cells (2,000 cells per well in six-well plates) were allowed to grow for 12 days before being fixed with methanol and stained with crystal violet. Data shown are representative of three individual experiments. Scale bar, 1 cm. Full size image To facilitate further investigation, we established Mel-FH and ME1007 sublines (Mel-FH.PIB5PA and ME1007.PIB5PA) conditionally expressing PIB5PA in response to 4-hydroxytamoxifen (4-OHT) [38] . The addition of 4-OHT readily induced PIB5PA, reduced pSer473-Akt and inhibited cell proliferation ( Fig. 3a and Supplementary Fig. S5 ). When 4-OHT was withdrawn, activation of Akt and cell proliferation rates were restored, which were associated with diminishing of induced PIB5PA ( Fig. 3b–d ). Furthermore, introduction of an active form of Akt (myr-Akt) into the Mel-FH.PIB5PA and ME1007.PIB5PA cells reversed 4-OHT-induced inhibition of proliferation ( Fig. 3e–g ) [39] . These results consolidate that PIB5PA negatively regulates melanoma cell proliferation by inhibiting PI3K/Akt signalling. As expected, introduction of myr-Akt promoted cell proliferation in parental ME1007 and Mel-FH cells ( Supplementary Fig. S6 ). 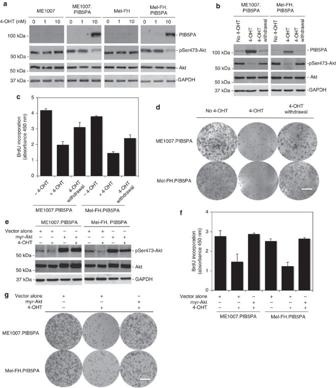Figure 3: PIB5PA-triggered inhibition of cell proliferation is due to inhibition of PI3K/Akt. (a) Mel-FH.PIB5PA and ME1007.PIB5PA cells that carried a lentiviral-based 4-OHT-responsive inducible gene expression system and their parental counterparts were exposed to 4-OHT at indicated concentrations for 24 h. Whole-cell lysates were subjected to western blot analysis. (b) Whole-cell lysates from Mel-FH.PIB5PA and ME1007.PIB5PA cells treated with 4-OHT (10 nM) for 24 h with or without withdrawal of 4-OHT for another 24 h were subjected to western blot analysis. (c) Mel-FH.PIB5PA and ME1007.PIB5PA cells treated with 4-OHT (10 nM) for 24 h with or without withdrawal of 4-OHT for another 48 h were subjected to proliferation assays using the BrdU incorporation method (n=3, mean±s.e.m.). (d) Mel-FH.PIB5PA and ME1007.PIB5PA cells were seeded onto six-well plates (2,000 cells per well) for 24 h before the addition of 4-OHT (10 nM). Seventy-two hours later, 4-OHT was withdrawn from representative wells. Cells were allowed to grow for another 9 days before being fixed with methanol and stained with crystal violet. Scale bar, 1 cm. (e) Mel-FH.PIB5PA and ME1007.PIB5PA cells were transiently transfected with vector alone or a myr-Akt construct. Twenty-four hours later, cells were treated with 4-OHT (10 nM) for a further 24 h. Whole-cell lysates were subjected to western blot analysis. (f) Mel-FH.PIB5PA and ME1007.PIB5PA cells were transiently transfected with vector alone or a myr-Akt construct. Twenty-four hours later, cells were treated with 4-OHT (10 nM) for a further 48 h before cell proliferation was measured by the BrdU incorporation method (n=3, mean±s.e.m.). (g) Mel-FH.PIB5PA and ME1007.PIB5PA cells were transfected with vector alone or a myr-Akt construct. Twenty-four hours later, viable cells (2,000 cells per well in six-well plates) were allowed to grow for a further 12 days before being fixed with methanol and stained with crystal violet. Scale bar, 1 cm. Figure 3: PIB5PA-triggered inhibition of cell proliferation is due to inhibition of PI3K/Akt. ( a ) Mel-FH.PIB5PA and ME1007.PIB5PA cells that carried a lentiviral-based 4-OHT-responsive inducible gene expression system and their parental counterparts were exposed to 4-OHT at indicated concentrations for 24 h. Whole-cell lysates were subjected to western blot analysis. ( b ) Whole-cell lysates from Mel-FH.PIB5PA and ME1007.PIB5PA cells treated with 4-OHT (10 nM) for 24 h with or without withdrawal of 4-OHT for another 24 h were subjected to western blot analysis. ( c ) Mel-FH.PIB5PA and ME1007.PIB5PA cells treated with 4-OHT (10 nM) for 24 h with or without withdrawal of 4-OHT for another 48 h were subjected to proliferation assays using the BrdU incorporation method ( n =3, mean±s.e.m.). ( d ) Mel-FH.PIB5PA and ME1007.PIB5PA cells were seeded onto six-well plates (2,000 cells per well) for 24 h before the addition of 4-OHT (10 nM). Seventy-two hours later, 4-OHT was withdrawn from representative wells. Cells were allowed to grow for another 9 days before being fixed with methanol and stained with crystal violet. Scale bar, 1 cm. ( e ) Mel-FH.PIB5PA and ME1007.PIB5PA cells were transiently transfected with vector alone or a myr-Akt construct. Twenty-four hours later, cells were treated with 4-OHT (10 nM) for a further 24 h. Whole-cell lysates were subjected to western blot analysis. ( f ) Mel-FH.PIB5PA and ME1007.PIB5PA cells were transiently transfected with vector alone or a myr-Akt construct. Twenty-four hours later, cells were treated with 4-OHT (10 nM) for a further 48 h before cell proliferation was measured by the BrdU incorporation method ( n =3, mean±s.e.m.). ( g ) Mel-FH.PIB5PA and ME1007.PIB5PA cells were transfected with vector alone or a myr-Akt construct. Twenty-four hours later, viable cells (2,000 cells per well in six-well plates) were allowed to grow for a further 12 days before being fixed with methanol and stained with crystal violet. Scale bar, 1 cm. Full size image We also tested the effect of another two 5-phosphatases, oculocerebrorenal syndrome of Lowe (OCRL) and SHIP2, on PI3K/Akt signalling. Strikingly, both OCRL and SHIP2 were expressed at higher levels in most melanoma cell lines compared with melanocytes ( Supplementary Fig. S7 ). Nonetheless, these 5-phosphatases did not appear to have a major role in regulating PI3K/Akt signalling, as small interfering RNA (siRNA) knockdown of OCRL or SHIP2 in melanoma cells expressing relatively high levels of the protein, or overexpression of OCRL or SHIP2 in those expressing relatively low levels of the protein, did not cause any noticeable change in pSer473-Akt levels, nor did it impinge on cell viability ( Supplementary Figs. S8 and S9 ). Deregulation of PIB5PA modulates tumour growth To investigate whether PIB5PA-mediated inhibition of PI3K/Akt has a role in suppression of melanocyte transformation, we knocked down PIB5PA in human adult epidermal melanocytes (HEMa-LP cells) with lentiviral transduction of PIB5PA short hairpin RNA (shRNA; Fig. 4a ). This caused anchorage-independent growth comparable to that observed with a PTEN shRNA ( Fig. 4c ). Knockdown of PIB5PA or PTEN also increased the proliferation rate of HEMa-LP cells and the effect of knockdown of PIB5PA could be reversed by cointroduction of a shRNA against Akt, indicating that it was mediated by activation of PI3K/Akt signalling ( Fig. 4e–g ). 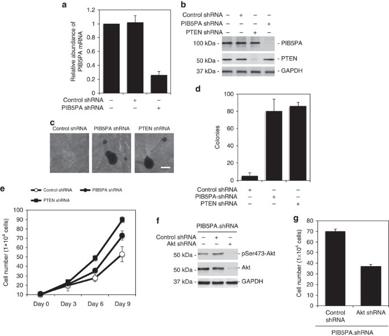Figure 4: Knockdown of PIB5PA results in anchorage-independent growth of melanocytes. (a) The PIB5PA mRNA expression levels in HEMa-LP melanocytes transduced with the control or PIB5PA shRNA by quantitative PCR (n=3, mean±s.e.m.). (b) Whole-cell lysates from HEMa-LP melanocytes transduced with the control or PIB5PA shRNA were subjected to western blot analysis. (c) Anchorage-independent growth assay of HEMa-LP melanocytes transduced with the control, PIB5PA or PTEN shRNA. Scale bar, 0.5 mm. (d) Quantification of anchorage-independent growth assay of HEMa-LP melanocytes transduced with the control, PIB5PA or PTEN shRNA as shown inc(n=3, mean±s.e.m.; Student’st-test; *P<0.05). (e) HEMa-LP melanocytes transduced with the control, PIB5PA or PTEN shRNA were counted on days 3, 6 and 9, using an automated cell counter (n=3, mean±s.e.m.). (f) HEMa-LP melanocytes transduced with the PIB5PA shRNA were cointroduced with the control or Akt shRNA. Twenty-four hours later, whole-cell lysates were subjected to western blot analysis. (g) HEMa-LP melanocytes transduced with the PIB5PA shRNA were cointroduced with the control or Akt shRNA. Ninety-six hours later, viable cells were counted in an automated cell counter (n=3, mean±s.e.m.). Figure 4: Knockdown of PIB5PA results in anchorage-independent growth of melanocytes. ( a ) The PIB5PA mRNA expression levels in HEMa-LP melanocytes transduced with the control or PIB5PA shRNA by quantitative PCR ( n =3, mean±s.e.m.). ( b ) Whole-cell lysates from HEMa-LP melanocytes transduced with the control or PIB5PA shRNA were subjected to western blot analysis. ( c ) Anchorage-independent growth assay of HEMa-LP melanocytes transduced with the control, PIB5PA or PTEN shRNA. Scale bar, 0.5 mm. ( d ) Quantification of anchorage-independent growth assay of HEMa-LP melanocytes transduced with the control, PIB5PA or PTEN shRNA as shown in c ( n =3, mean±s.e.m. ; Student’s t -test; * P <0.05). ( e ) HEMa-LP melanocytes transduced with the control, PIB5PA or PTEN shRNA were counted on days 3, 6 and 9, using an automated cell counter ( n =3, mean±s.e.m.). ( f ) HEMa-LP melanocytes transduced with the PIB5PA shRNA were cointroduced with the control or Akt shRNA. Twenty-four hours later, whole-cell lysates were subjected to western blot analysis. ( g ) HEMa-LP melanocytes transduced with the PIB5PA shRNA were cointroduced with the control or Akt shRNA. Ninety-six hours later, viable cells were counted in an automated cell counter ( n =3, mean±s.e.m.). Full size image We exploited tumour growth of ME1007.PIB5PA and Mel-FH.PIB5PA cells subcutaneously transplanted into nu/nu mice treated with 4-OHT or the vehicle control, to determine the functional significance of expression of PIB5PA in melanoma growth in vivo . In this model, treatment with 4-OHT caused significant retardation of tumour growth in vivo ( Fig. 5a and Supplementary Fig. S10 ). This was associated with induction of PIB5PA, suppression of activation of Akt and upregulation of p27 ( Fig. 5c and Supplementary Fig. S10 ). The role of inhibition of PI3K/Akt signalling in PIB5PA-mediated suppression of melanoma tumourigenesis was confirmed by transplanting ME1007.PIB5PA cells cointroduced with myr-Akt into nu/nu mice. This demonstrated that expression of myr-Akt effectively restored tumour growth that was associated with resuppression of p27 in mice treated with 4-OHT ( Fig. 5d–g ). 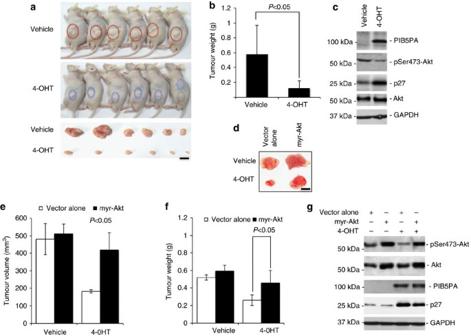Figure 5: Overexpression of PIB5PA reduces melanoma growth in a xenograft mouse model. (a) Viable ME1007.PIB5PA cells (1 × 107), with or without pretreatment with 4-OHT (10 nM) for 36 h, were subcutaneously injected into flanks of nu/nu mice. Two days later, mice were administered with either vehicle (DMSO;n=6) or 4-OHT (10 nM g−1;n=6) via intraperitoneal injections every 3 days. Mice were killed and tumours were collected at 36 days after melanoma cell injection. Data shown are representative of three individual experiments. Scale bar, 5 mm. (b) Comparison of weight of tumours from animals treated with 4-OHT with those treated with vehicle control (n=6, mean±s.e.m.; Student’st-test; *P<0.05). (c) Whole-cell lysates of crude tumour tissues were subjected to western blot analysis. Data shown are representative of three individual western blot analyses of randomly selected tumour samples from mice with or without treatment with 4-OHT. (d) Representative tumours generated by ME1007.PIB5PA cells with or without cotransduction with myr-Akt in nu/nu mice with or without treatment with 4-OHT as stated ina. Scale bar, 5 mm. (e,f) Comparison of volume (e) and weight (f) of tumours generated by ME1007.PIB5PA cells with or without cotransduced myr-Akt in nu/nu mice with or without treatment with 4-OHT as stated ina(n=6, mean±s.e.m.; Student’st-test; *P<0.05). (g) Whole-cell lysates of crude tumour tissues from tumours generated by ME1007.PIB5PA cells with or without cotransduced with myr-Akt in nu/nu mice with or without treatment with 4-OHT as stated ina. Data shown are representative of three individual experiments. Figure 5: Overexpression of PIB5PA reduces melanoma growth in a xenograft mouse model. ( a ) Viable ME1007.PIB5PA cells (1 × 10 7 ), with or without pretreatment with 4-OHT (10 nM) for 36 h, were subcutaneously injected into flanks of nu/nu mice. Two days later, mice were administered with either vehicle (DMSO; n =6) or 4-OHT (10 nM g −1 ; n =6) via intraperitoneal injections every 3 days. Mice were killed and tumours were collected at 36 days after melanoma cell injection. Data shown are representative of three individual experiments. Scale bar, 5 mm. ( b ) Comparison of weight of tumours from animals treated with 4-OHT with those treated with vehicle control ( n =6, mean±s.e.m. ; Student’s t -test; * P <0.05). ( c ) Whole-cell lysates of crude tumour tissues were subjected to western blot analysis. Data shown are representative of three individual western blot analyses of randomly selected tumour samples from mice with or without treatment with 4-OHT. ( d ) Representative tumours generated by ME1007.PIB5PA cells with or without cotransduction with myr-Akt in nu/nu mice with or without treatment with 4-OHT as stated in a . Scale bar, 5 mm. ( e , f ) Comparison of volume ( e ) and weight ( f ) of tumours generated by ME1007.PIB5PA cells with or without cotransduced myr-Akt in nu/nu mice with or without treatment with 4-OHT as stated in a ( n =6, mean±s.e.m. ; Student’s t -test; * P <0.05). ( g ) Whole-cell lysates of crude tumour tissues from tumours generated by ME1007.PIB5PA cells with or without cotransduced with myr-Akt in nu/nu mice with or without treatment with 4-OHT as stated in a . Data shown are representative of three individual experiments. Full size image PIB5PA and PTEN cooperatively suppress PI3K signalling We confirmed the role of PIB5PA in inhibition of PI3K/Akt signalling in serum-starved ME1007.PIB5PA and Mel-FH.PIB5PA cells. The levels of pSer473-Akt were markedly lower in the cells concomitantly exposed to 4-OHT than those without the addition of 4-OHT ( Fig. 6a ). When subsequently stimulated with epidermal growth factor (EGF), the kinetics of Akt activation was decelerated and the magnitude reduced in the cells overexpressing PIB5PA ( Fig. 6a and Supplementary Fig. S11 ). As anticipated, transfection of PTEN also resulted in the inhibition of activation of Akt; however, the kinetics of Akt activation triggered by EGF in these transfected cells was similar to that of the control cells ( Fig. 6c and Supplementary Fig. S11 ). The inhibitory effect on Akt activation was further enhanced when a PTEN construct was introduced into ME1007.PIB5PA and Mel-FH.PIB5PA cells followed by treatment with 4-OHT ( Fig. 6e ). 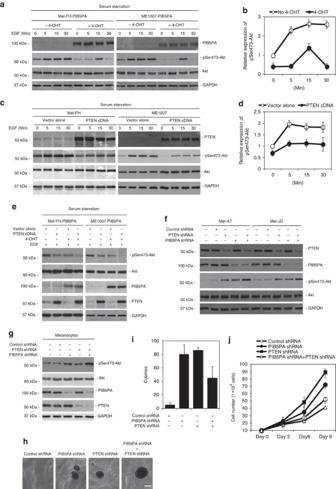Figure 6: PIB5PA and PTEN cooperatively regulate the activation of Akt. (a) Mel-FH.PIB5PA and ME1007.PIB5PA cells were serum-starved for 16 h in the presence or absence of 4-OHT (10 nM) before stimulation with EGF (100 nM) for indicated periods. Whole-cell lysates were subjected to western blot analysis. (b) Quantification of levels of pSer473-Akt in Mel-FH.PIB5PA cells as shown ina, which were normalized to those of total Akt (n=3, mean±s.e.m.). (c) Mel-FH and ME1007 cells were transiently transfected with a PTEN construct. Twenty-four hours later, cells were serum-starved for 16 h, followed by stimulation with EGF (100 nM) for indicated periods. Whole-cell lysates were subjected to western blot analysis. (d) Quantification of levels of pSer473-Akt in Mel-FH cells as shown inc, which were normalized to those of total Akt (n=3, mean±s.e.m.). (e) Mel-FH.PIB5PA and ME1007.PIB5PA cells were transiently transfected with a PTEN construct. Twenty-four hours later, cells were switched into serum-free medium with or without 4-OHT (10 nM) for a further 16 h before the addition of EGF (100 nM) for 15 min. Whole-cell lysates were subjected to western blot analysis. (f) Mel-AT and Mel-JD were transfected with the control, PIB5PA, PTEN or PIB5PA plus PTEN siRNA. Twenty-four hours later, whole-cell lysates were subjected to western blot analysis. (g) HEMa-LP melanocytes were transfected with the control, PIB5PA, PTEN or PIB5PA plus PTEN siRNA. Twenty-four hours later, whole-cell lysates were subjected to western blot analysis. (h) Anchorage-independent growth assay of HEMa-LP melanocytes transduced with the control, PIB5PA, PTEN or PIB5PA plus PTEN shRNA. Data shown are representative of three individual experiments. Scale bar, 0.5 mm. (i) Quantification of anchorage-independent growth assay of HEMa-LP melanocytes transduced with the control, PIB5PA, PTEN or PIB5PA plus PTEN shRNA as shown inh(n=3, mean±s.e.m.). (j) HEMa-LP melanocytes transduced with the control, PIB5PA, PTEN or PIB5PA plus PTEN shRNA as shown inhwere counted on days 3, 6 and 9, using an automated cell counter (n=3, mean±s.e.m.). Figure 6: PIB5PA and PTEN cooperatively regulate the activation of Akt. ( a ) Mel-FH.PIB5PA and ME1007.PIB5PA cells were serum-starved for 16 h in the presence or absence of 4-OHT (10 nM) before stimulation with EGF (100 nM) for indicated periods. Whole-cell lysates were subjected to western blot analysis. ( b ) Quantification of levels of pSer473-Akt in Mel-FH.PIB5PA cells as shown in a , which were normalized to those of total Akt ( n =3, mean±s.e.m.). ( c ) Mel-FH and ME1007 cells were transiently transfected with a PTEN construct. Twenty-four hours later, cells were serum-starved for 16 h, followed by stimulation with EGF (100 nM) for indicated periods. Whole-cell lysates were subjected to western blot analysis. ( d ) Quantification of levels of pSer473-Akt in Mel-FH cells as shown in c , which were normalized to those of total Akt ( n =3, mean±s.e.m.). ( e ) Mel-FH.PIB5PA and ME1007.PIB5PA cells were transiently transfected with a PTEN construct. Twenty-four hours later, cells were switched into serum-free medium with or without 4-OHT (10 nM) for a further 16 h before the addition of EGF (100 nM) for 15 min. Whole-cell lysates were subjected to western blot analysis. ( f ) Mel-AT and Mel-JD were transfected with the control, PIB5PA, PTEN or PIB5PA plus PTEN siRNA. Twenty-four hours later, whole-cell lysates were subjected to western blot analysis. ( g ) HEMa-LP melanocytes were transfected with the control, PIB5PA, PTEN or PIB5PA plus PTEN siRNA. Twenty-four hours later, whole-cell lysates were subjected to western blot analysis. ( h ) Anchorage-independent growth assay of HEMa-LP melanocytes transduced with the control, PIB5PA, PTEN or PIB5PA plus PTEN shRNA. Data shown are representative of three individual experiments. Scale bar, 0.5 mm. ( i ) Quantification of anchorage-independent growth assay of HEMa-LP melanocytes transduced with the control, PIB5PA, PTEN or PIB5PA plus PTEN shRNA as shown in h ( n =3, mean±s.e.m.). ( j ) HEMa-LP melanocytes transduced with the control, PIB5PA, PTEN or PIB5PA plus PTEN shRNA as shown in h were counted on days 3, 6 and 9, using an automated cell counter ( n =3, mean±s.e.m.). Full size image To further investigate the interaction between PIB5PA and PTEN in the regulation of activation of PI3K/Akt signalling, we knocked down PIB5PA and PTEN simultaneously in Mel-AT and Mel-JD cells that expressed relatively high levels of the proteins. Co-knockdown of PIB5PA and PTEN resulted in further increases in activation of Akt in comparison with knockdown of PIB5PA or PTEN alone (Fig. 6f ), suggesting that the regulatory effects of PIB5PA and PTEN on activation of PI3K/Akt signalling are not redundant. Similarly, the co-knockdown of PIB5PA and PTEN led to enhanced Akt activation and enlarged anchorage-independent colonies compared with the knockdown of PIB5PA or PTEN individually in HEMa-LP melanocytes (Fig. 6g ). However, the numbers of colonies formed by dual knockdown cells appeared fewer than those formed by the PIB5PA or PTEN single knockdown cells ( Fig. 6i ), and the proliferation rate of the double knockdown cells were decreased ( Fig. 6j ). These results indicate that loss of both PIB5PA and PTEN impairs melanocyte proliferation. Nevertheless, a proportion of cells with PIB5PA and PTEN simultaneously inhibited acquire enhanced proliferative potential that would promote cell transformation. Genomic alterations of the PIB5PA gene in melanoma cells To determine whether genomic alterations of the PIB5PA gene INPP5J are involved in its downregulation in melanoma cells, we analysed a previously published data set of 76 melanoma cell lines assessed with 317 K whole-genome single-nucleotide polymorphism arrays [40] . Although the whole-arm copy number losses occurred for chromosome 22q (where INPP5J maps to 22q12.2) in 6%, whole-arm copy number gain was found in another 29% of the melanoma cell lines. No regional loss of heterozygosity (LOH) at 22q12 was detected that spanned across INPP5J (31,518,717–31,530,683 bp) [40] . By using of quantitative PCR analysis of genomic DNA, we identified the reduction of INPP5J copy number in 2 of the 10 melanoma cell lines (20%), and 3 of the 20 fresh melanoma isolates (15%) of the cohort used in this study ( Fig. 1c and Supplementary Fig. S12 ). In keeping with the previous report [40] , the INPP5J copy number gain occurred in 3 of the 10 melanoma cell lines (30%) and 5 of the 20 fresh melanoma isolates (25%; Supplementary Fig. S12 ). Strikingly, neither ME1007 nor Mel-FH, which expressed the lowest levels of the PIB5PA transcript and protein, had INPP5J copy number loss ( Fig. 1f and Supplementary Fig. S12 ). Moreover, no mutation was detected in all but 1 melanoma cell line that carried a G for A substitution at exon 7 by exon sequencing of all the 13 exons of INPP5J ( Supplementary Fig. S13 ). Collectively, these results indicate that although gene copy number reduction is responsible for downregulation of PIB5PA in a proportion of cases, mechanisms other than genomic alterations may be the main cause of suppression of PIB5PA in melanoma. PIB5PA expression is suppressed by histone hypoacetylation Promoter hypermethylation is a common mechanism of PTEN inactivation in human melanoma [41] . We therefore examined whether a similar mechanism is involved in the suppression of PIB5PA in melanoma cells. The methylation inhibitor 5-aza-2′-deoxycytidine triggered an increase in PTEN, but not PIB5PA ( Fig. 7a and Supplementary Fig. S14 ). In contrast, the HDAC inhibitor SAHA markedly increased PIB5PA, but not PTEN ( Fig. 7c and Supplementary Fig. S14 ), suggesting that PIB5PA is epigenetically suppressed by histone hypoacetylation. In support, SAHA increased the INPP5J promoter activity as demonstrated in Mel-FH and ME1007 cells transfected with luciferase reporter plasmids of the INPP5J core promoter containing sequences between −2,016 and +114 (pGL3- INPP5J -(−2,016/+114); numbers relative to the transcription start site; Fig. 7e ). 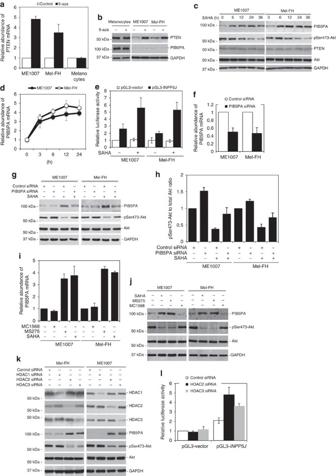Figure 7: PIB5PA is suppressed by HDAC2 and HDAC3 in melanoma cells. (a) Total RNA from ME1007 and Mel-FH cells treated with 5-aza (5-aza-2′-deoxycytidine; 10 μM) for 96 h were subjected to quantitative PCR (qPCR) analysis (n=3, mean±s.e.m.). (b) Whole-cell lysates from HEMa-LP melanocytes, and ME1007 and Mel-FH melanoma cells treated with 5-aza (10 μM) for 96 h were subjected to western blot analysis. (c) Whole-cell lysates from ME1007 and Mel-FH cells treated with SAHA (4 μM) for indicated periods were subjected to western blot analysis. (d) Total RNA from ME1007 and Mel-FH cells treated with SAHA (4 μM) for indicated periods were subjected to qPCR analysis (n=3, mean±s.e.m.). (e) ME1007 and Mel-FH cells were transiently transfected with the pGL3-basic-based reporter constructs, pGL3-vector and pGL3-INPP5Jcore promoter (pGL3-INPP5J−2,016/+114), respectively. Twenty-four hours later, cells were treated with SAHA (4 μM) for a further 24 h, followed by measurement of the luciferase activity (n=3, mean±s.e.m.). (f) ME1007 and Mel-FH cells were transfected with the control or PIB5PA siRNA. Twenty-four hours later, total RNA was subjected qPCR analysis of PIB5PA mRNA expression (n=3, mean±s.e.m.). (g) ME1007 and Mel-FH cells were transfected with the control or PIB5PA siRNA. Twenty-four hours later, cells were treated with SAHA (4 μM) for a further 24 h. Whole-cell lysates were subjected to western blot analysis. (h) Quantification of pSer473-Akt normalized to total Akt levels as shown ing(n=3, mean±s.e.m.). (i) Total RNA from ME1007 and Mel-FH cells treated with MC1568 (5 μM), MS275 (5 μM) and SAHA (4 μM), respectively, for 24 h was subjected to qPCR analysis of PIB5PA mRNA. The relative abundance of PIB5PA mRNA in cells treated with MC1568, MS275 or SAHA was normalized to that in cells without treatment (n=3, mean±s.e.m.). (j) Whole-cell lysates from ME1007 and Mel-FH cells treated with MC1568 (5 μM), MS275 (5 μM) and SAHA (4 μM), respectively, for 24 h were subjected to western blot analysis. (k) Whole-cell lysates from ME1007 and Mel-FH cells transfected with the control, HDAC1, HDAC2 or HDAC3 siRNA were subjected to western blot analysis. (l) ME1007 cells were cotransfected with the control, HDAC2 or HDAC3 siRNA, and pGL3-INPP5J-(−2,016/+114). Luciferase activity was measured 24 h after transfection (n=3, mean±s.e.m.). Figure 7: PIB5PA is suppressed by HDAC2 and HDAC3 in melanoma cells. ( a ) Total RNA from ME1007 and Mel-FH cells treated with 5-aza (5-aza-2′-deoxycytidine; 10 μM) for 96 h were subjected to quantitative PCR (qPCR) analysis ( n =3, mean±s.e.m.). ( b ) Whole-cell lysates from HEMa-LP melanocytes, and ME1007 and Mel-FH melanoma cells treated with 5-aza (10 μM) for 96 h were subjected to western blot analysis. ( c ) Whole-cell lysates from ME1007 and Mel-FH cells treated with SAHA (4 μM) for indicated periods were subjected to western blot analysis. ( d ) Total RNA from ME1007 and Mel-FH cells treated with SAHA (4 μM) for indicated periods were subjected to qPCR analysis ( n =3, mean±s.e.m.). ( e ) ME1007 and Mel-FH cells were transiently transfected with the pGL3-basic-based reporter constructs, pGL3-vector and pGL3- INPP5J core promoter (pGL3- INPP5J −2,016/+114), respectively. Twenty-four hours later, cells were treated with SAHA (4 μM) for a further 24 h, followed by measurement of the luciferase activity ( n =3, mean±s.e.m.). ( f ) ME1007 and Mel-FH cells were transfected with the control or PIB5PA siRNA. Twenty-four hours later, total RNA was subjected qPCR analysis of PIB5PA mRNA expression ( n =3, mean±s.e.m.). ( g ) ME1007 and Mel-FH cells were transfected with the control or PIB5PA siRNA. Twenty-four hours later, cells were treated with SAHA (4 μM) for a further 24 h. Whole-cell lysates were subjected to western blot analysis. ( h ) Quantification of pSer473-Akt normalized to total Akt levels as shown in g ( n =3, mean±s.e.m.). ( i ) Total RNA from ME1007 and Mel-FH cells treated with MC1568 (5 μM), MS275 (5 μM) and SAHA (4 μM), respectively, for 24 h was subjected to qPCR analysis of PIB5PA mRNA. The relative abundance of PIB5PA mRNA in cells treated with MC1568, MS275 or SAHA was normalized to that in cells without treatment ( n =3, mean±s.e.m.). ( j ) Whole-cell lysates from ME1007 and Mel-FH cells treated with MC1568 (5 μM), MS275 (5 μM) and SAHA (4 μM), respectively, for 24 h were subjected to western blot analysis. ( k ) Whole-cell lysates from ME1007 and Mel-FH cells transfected with the control, HDAC1, HDAC2 or HDAC3 siRNA were subjected to western blot analysis. ( l ) ME1007 cells were cotransfected with the control, HDAC2 or HDAC3 siRNA, and pGL3- INPP5J -(−2,016/+114). Luciferase activity was measured 24 h after transfection ( n =3, mean±s.e.m.). Full size image Notably, SAHA also induced a decrease in Akt activation that was mediated at least in part by increased PIB5PA, in that inhibition of the latter attenuated the effect of SAHA on pSer473-Akt ( Fig. 7f–h ). Suppression of PIB5PA expression by histone hypoacetylation seemed to be a general yet specific mechanism of regulation of PI3K/Akt signalling in melanoma as shown by upregulation of PIB5PA by SAHA in a panel of melanoma cell lines, but not in melanocytes ( Supplementary Fig. S14 ). The functional consequence of SAHA-triggered upregulation of PIB5PA was demonstrated by the inhibition of SAHA-induced reduction in cell viability with knockdown of PIB5PA ( Supplementary Fig. S15 ), which was recapitulated by introducing myr-Akt into the cells ( Supplementary Fig. S15 ). Similar to SAHA, the HDAC inhibitor sodium butyrate that selectively inhibits class I and class IIa HDACs also upregulated PIB5PA in melanoma cells (Supplementary Fig. S14) [42] , suggesting that suppression of PIB5PA by histone hypoacetylation is mediated by one or more HDACs of these classes. To elucidate the HDAC(s) responsible, we treated Mel-FH and ME1007 cells, respectively, with the HDAC inhibitors MS275 that preferentially inhibits the class I HDACs, HDAC1, -2 and -3, and MC1568 that specifically inhibits Class IIa HDACs [42] . Although MC1568 had no effect on PIB5PA mRNA expression, MS275 upregulated PIB5PA and downregulated pSer473-Akt ( Fig. 7i ). Furthermore, knockdown of HDAC2 or -3, but not of HDAC1, recapitulated the effect of MS275 ( Fig. 7k ), pinpointing HDAC2 and -3 as the major HDACs responsible for suppression of PIB5PA in melanoma cells. This was further supported by inhibition of the INPP5J promoter activity when HDAC2 or -3 was knocked down ( Fig. 7l ). HDAC2 and -3 repress INPP5J transcription by binding Sp1 To elucidate the mechanisms involved in regulation of PIB5PA by HDAC2 and -3 in melanoma cells, we sought to determine the active region of the INPP5J promoter in response to MS275. As plasmid reporter systems had been shown to be useful tools in examining the effects of inhibition of HDACs on promoter activity of target genes [43] , [44] , we analysed the responses of a series of incremental deletion reporter constructs contained in the −2,016/+114 region to MS275 ( Fig. 8a ). MS275 increased the transcriptional activity in all the constructs, but pGL3- INPP5J -(−116/+114). The shortest MS275-responsive fragment was pGL3- INPP5J -(−516/+114; Fig. 8b and Supplementary Fig. S16 ). Therefore, the region between −516 and −116 is required for transcriptional upregulation of PIB5PA by inhibition of HDAC2 and -3. This was confirmed by siRNA knockdown of HDAC2 or -3 ( Fig. 8c and Supplementary Fig. S16 ). 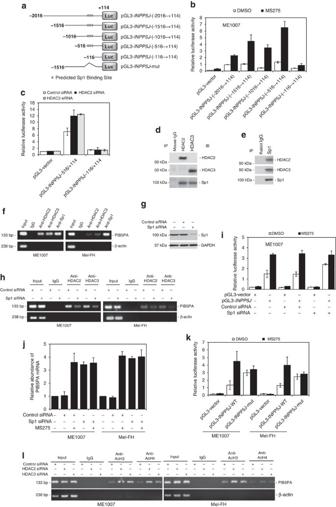Figure 8: HDAC2 and HDAC3 repressINPP5Jthrough binding to Sp1. (a) A schematic illustration of construction of a luciferase reporter constructs. (b) ME1007 cells were transiently transfected with indicated pGL3-basic-based reporter constructs. Twenty-four hours later, cells were treated with MS275 (5 μM) for a further 24 h, followed by measurement of the luciferase activity (n=3, mean±s.e.m.). (c) ME1007 cells were cotransfected with the control, HDAC2 or HDAC3 siRNA, and indicated pGL3-basic-based reporter constructs. Luciferase activity was measured 24 h after transfection (n=3, mean±s.e.m.). (d,e) Coimmunoprecipitation assays showing physical association of HDAC2 and HDAC3 with Sp1 in ME1007 cells. (f) Formaldehyde-crosslinked chromatin of ME1007 and Mel-FH cells was subjected to immunoprecipitation with antibodies against HDAC2, HDAC3 or Sp1. The precipitates were subjected to PCR amplification using primers directed to the −516/−383 (133 bp) fragment of theINPP5Jpromoter. Data shown are representative of three individual experiments. (g) Western blotting showing siRNA knockdown of Sp1 in ME1007 cells. (h) ChIP assays showing knockdown of Sp1 abolished the association of HDAC2 and HDAC3 with the INPP5J promoter. (i) ME1007 cells were cotransfected with the control or Sp1 siRNA and pGL3-vector or pGL3-INPP5J-(−2,016/+144) (pGL3-INPP5J). Twenty-four hours later, cells were treated with MS275 (5 μM) for a further 24 h, followed by measurement of the luciferase activity (n=3, mean±s.e.m.). (j) quantitative PCR analysis showing that siRNA knockdown of Sp1 elevated the levels of PIB5PA mRNA, which could not be further increased by MS275 (n=3, mean±s.e.m.). (k) ME1007 and Mel-FH cells were transiently transfected with the pGL3-basic-based reporter constructs, pGL3-vector, pGL3-INPP5J-(−1,516/+144) (pGL3-INPP5J-WT) and a reporter with the Sp1 binding site-enriched fragment deleted as shown ina(pGL3-INPP5J-mutant), respectively. Twenty-four hours later, cells were treated with MS275 (5 μM) for a further 24 h, followed by measurement of the luciferase activity (n=3, mean±s.e.m.). (l) ChIP assays showing increased acetylation of the H3 and H4 histone subunits associated with INPP5J promoter (−516/−383) when HDAC2 or HDAC3 was knocked down. Figure 8: HDAC2 and HDAC3 repress INPP5J through binding to Sp1. ( a ) A schematic illustration of construction of a luciferase reporter constructs. ( b ) ME1007 cells were transiently transfected with indicated pGL3-basic-based reporter constructs. Twenty-four hours later, cells were treated with MS275 (5 μM) for a further 24 h, followed by measurement of the luciferase activity ( n =3, mean±s.e.m.). ( c ) ME1007 cells were cotransfected with the control, HDAC2 or HDAC3 siRNA, and indicated pGL3-basic-based reporter constructs. Luciferase activity was measured 24 h after transfection ( n =3, mean±s.e.m.). ( d , e ) Coimmunoprecipitation assays showing physical association of HDAC2 and HDAC3 with Sp1 in ME1007 cells. ( f ) Formaldehyde-crosslinked chromatin of ME1007 and Mel-FH cells was subjected to immunoprecipitation with antibodies against HDAC2, HDAC3 or Sp1. The precipitates were subjected to PCR amplification using primers directed to the −516/−383 (133 bp) fragment of the INPP5J promoter. Data shown are representative of three individual experiments. ( g ) Western blotting showing siRNA knockdown of Sp1 in ME1007 cells. ( h ) ChIP assays showing knockdown of Sp1 abolished the association of HDAC2 and HDAC3 with the INPP5J promoter. ( i ) ME1007 cells were cotransfected with the control or Sp1 siRNA and pGL3-vector or pGL3- INPP5J -(−2,016/+144) (pGL3- INPP5J ). Twenty-four hours later, cells were treated with MS275 (5 μM) for a further 24 h, followed by measurement of the luciferase activity ( n =3, mean±s.e.m.). ( j ) quantitative PCR analysis showing that siRNA knockdown of Sp1 elevated the levels of PIB5PA mRNA, which could not be further increased by MS275 ( n =3, mean±s.e.m.). ( k ) ME1007 and Mel-FH cells were transiently transfected with the pGL3-basic-based reporter constructs, pGL3-vector, pGL3- INPP5J -(−1,516/+144) (pGL3- INPP5J-WT ) and a reporter with the Sp1 binding site-enriched fragment deleted as shown in a (pGL3- INPP5J -mutant), respectively. Twenty-four hours later, cells were treated with MS275 (5 μM) for a further 24 h, followed by measurement of the luciferase activity ( n =3, mean±s.e.m.). ( l ) ChIP assays showing increased acetylation of the H3 and H4 histone subunits associated with INPP5J promoter (−516/−383) when HDAC2 or HDAC3 was knocked down. Full size image The −516/−116 region of the INPP5J promoter is enriched of consensus binding sites for the transcription factor Sp1 ( Supplementary Fig. S17 ). The latter can form transcriptional repressing complexes with HDACs at many gene promoters [45] , [46] , [47] . Indeed, HDAC2 and -3 were physically associated with Sp1 in ME1007 and Mel-FH cells ( Fig. 8d and Supplementary Fig. S18 ). In addition, chromatin immunoprecipitation (ChIP) assays demonstrated the association of HDAC2 and -3 and Sp1 with the INPP5J promoter in the cells ( Fig. 8f ). However, no such association was detected in HEMn-LP melanocytes ( Supplementary Fig. S19 ). The association between HDAC2 and -3 and the INPP5J promoter in melanoma cells was abolished when Sp1 was knocked down ( Fig. 8g and Supplementary Fig. S20 ). Furthermore, knockdown of Sp1 recapitulated the effect of MS275 on the transcriptional activity of the INPP5J promoter ( Fig. 8i and Supplementary Fig. S20 ). On the other hand, MS275 did not trigger any further increase in the activity in cells with Sp1 knocked down ( Fig. 8i and Supplementary Fig. S20 ). When the Sp1 binding sites at the −516/−116 region were deleted, the transcriptional activity of the INPP5J promoter was similarly elevated, which could not be further increased by MS275 ( Fig. 8k ). These results indicate that binding of Sp1 to its binding sites at the −516/−116 region is required for repression of the INPP5J transcription by HDAC2 and -3 in melanoma cells. This was further demonstrated by increased acetylation of the H3 and H4 histone subunits associated with the region when HDAC2 or HDAC3 was knocked down ( Fig. 8l ). In contrast, knockdown of HDAC2 or HDAC3 did not alter the relatively high acetylation levels of the H3 and H4 subunits associated with the region ( Supplementary Fig. S21 ). In this report, we present evidence that the 5-phosphatase PIB5PA has an important tumour suppressive role by inhibiting PI3K/Akt signalling in melanoma ( Supplementary Fig. S22 ). Although its expression is commonly reduced or lost in melanoma cells in vitro and in vivo , introduction of exogenous PIB5PA resulted in decreased activation of Akt, which led to inhibition of proliferation and survival of melanoma cells in vitro , and retardation in melanoma tumour growth in a xenograft mouse model. On the other hand, knockdown of PIB5PA in melanocytes resulted in increased cell proliferation and anchorage-independent growth, similar to knockdown of PTEN. Our results also reveal that histone hypoacetylation mediated by HDAC2 and -3 through binding to the transcription factor Sp1 at the PIB5PA promoter is a common mechanism of suppressing PIB5PA in melanoma. Both the 3-phosphatase PTEN and 5-phosphatases can hydrolyse PI(3,4,5)P 3 ; the latter has been shown in many studies to be the most efficient phospholipid product of PI3K in activation of Akt, and is essential in PI3K-mediated oncogenic transformation [21] , [24] . However, only PTEN has been established as a tumour suppressor, whereas the role of 5-phosphatases in the pathogenesis of cancer remains controversial. This likely relates to the fact that hydrolysis of the phosphate group from the 5-position of PI(3,4,5)P 3 results in PI(3,4)P 2 , which can also recruit substrates, including Akt, leading to its activation [31] , [32] . Nevertheless, a number of 5-phosphatases, such as SHIP and SHIP2, have been demonstrated to have a role in suppressing PI3K/Akt signalling in various types of cancer cells [22] , [23] , [24] . Our results showing that overexpression of PIB5PA efficiently inhibits activation of Akt, whereas knockdown of PIB5PA promotes Akt activation, reveal a suppressive role of this 5-phosphatase in controlling PI3K/Akt signalling in melanoma cells. In contrast, we did not observe a similar role of another two 5-phosphatses, OCRL and SHIP2. Nevertheless, whether additional 5-phosphatases are involved in regulating PI3K/Akt signalling in melanoma cells needs further investigation. It is likely that various 5-phosphatases may regulate PI3K/Akt signalling in a highly cell type-specific manner. In this regard, it is noteworthy that functions of OCRL and SHIP2 are regulated by their post-translational modifications, such as phosphorylation or ubiquitination, subcellular localization and interactions with protein binding partners [48] , [49] . Consistent with its established role, overexpression of PTEN also resulted in inhibition of Akt activation in melanoma cells in response to EGF stimulation, but the magnitude of inhibition was not as great as that occurred with overexpression of PIB5PA. Nevertheless, although PTEN-triggered inhibition was steady, activation of Akt in melanoma cells overexpressing PIB5PA rebounded transiently. This suggests that PTEN and PIB5PA have similar yet distinct effects on regulating PI3K/Akt signalling. The rebound in Akt activation in PIB5PA-overexpressing cells is presumably due to generation of PI(3,4)P 2 (refs 31 , 32 ). Notably, co-overexpression of PIB5PA and PTEN resulted in further inhibition of Akt activation, indicating that these phosphatases cooperatively suppress PI3K/Akt signalling. In line with this, co-knockdown of PIB5PA and PTEN caused a further increase in activation of Akt in melanoma cells and melanocytes. Strikingly, dual knockdown of PIB5PA and PTEN resulted in inhibition of melanocyte proliferation and reduced numbers of anchorage-independent colonies, suggesting that, such as the coinhibition of INPP4B and PTEN, simultaneous inhibition of PIB5PA and PTEN may trigger senescence as a consequence of superactivation of PI3K/Akt signalling [29] . Although p53 is critical for induction of senescence by coinhibition of INPP4B and PTEN in other cell types [29] , pRb is the dominant effector of oncogene-induced melanocyte senescence [50] . Regardless, our results indicate that a proportion of melanocytes with PIB5PA and PTEN simultaneously inhibited can evade senescence and acquire proliferation advantages as shown by enlarged anchorage-independent colonies. Genetic alterations such as gene copy number reduction and LOH contribute to loss of PTEN in melanoma [35] , [36] , [51] . Our results, along with others’, indicate that INPP5J copy number reduction is responsible for downregulation of PIB5PA in a small proportion of melanomas, although LOH and other mutations of INPP5J seem uncommon [40] . Remarkably, consistent with the previous finding that whole-arm copy number gain occurred for chromosome 22q in 29% melanoma cell lines [40] , we detected increased INPP5J copy number in a relatively large proportion of melanoma cell lines (30%) and fresh melanoma isolates (25%), indicating that PIB5PA may be suppressed by an epigenetic mechanism(s) in the majority of melanomas. Indeed, although DNA methylation has a role in inhibition of PTEN [40] , we identified histone hypoacetylation mediated by HDAC2 and -3 as a common mechanism in downregulation of PIB5PA in melanoma. These data are in agreement with the notion that melanoma cells have evolved multiple complementary mechanisms to ensure that biological advantages can be achieved through activation of PI3K/Akt signalling [1] , [2] , and support a tumour suppressive role of PIB5PA in melanoma. Transcriptional repression of gene expression by histone hypoacetylation involves recruitment of the HDACs to gene promoters [42] , [45] , [46] , [47] . Consistently, we found that HDAC2 and -3 were associated with a region of the INPP5J promoter that was responsive to their inhibition through binding to the transcription factor Sp1. The latter has also been shown to form transcriptional repressing complexes with HDACs at many gene promoters [45] , [46] , [47] . HDAC2 and -3 are overexpressed, and contribute to development and progression of various cancers [42] , [45] , [47] . The expression of Sp1 is also upregulated in a number of malignant tumours [52] . Although it remains unknown whether HDAC2 and -3 and Sp1 are similarly increased in melanoma, our results clearly demonstrate that they have an important role in suppressing PIB5PA, leading to increased activation of PI3K/Akt signalling in melanoma cells. The tumour suppressive role of PIB5PA in melanoma is echoed by its reduced expression in melanoma cells in vivo . The significant decrease in PIB5PA levels in primary melanomas compared with nevi suggests that downregulation of PIB5PA, similar to loss of PTEN, is an early event during melanomagenesis [53] , [54] . However, there was no overall correlation between the levels of PIB5PA expression and Akt activation, reiterating that PI3K/Akt signalling is regulated by multiple mechanisms [1] , [2] . Of interest, the levels of PIB5PA and PTEN were significantly correlated, and loss of both was associated with particularly high levels of Akt activation in fresh melanoma isolates, suggesting that consistent with the finding in melanoma cell lines, downregulation of PIB5PA and PTEN may cooperatively promote activation of PI3K/Akt signalling in vivo , and that melanomas deficient in both PIB5PA and PTEN may be more profoundly dependent on survival advantages afforded by activation of the pathway. However, a similar association was not observed in studies on TMAs. This discrepancy may be related to variations in the sensitivity and specificity of different techniques in detection of protein expression. Irrespectively, the results from this study identify an important tumour suppressive role of PIB5PA in melanoma, and suggest that PIB5PA deficiency with or without concurrent reduction in PTEN may identify a subset of melanomas that are most likely susceptible to inhibition of the PI3K/Akt pathway. In addition, targeting HDAC2 and -3 may further enhance the therapeutic efficacy. Cell culture and human tissues Human melanoma cell lines described previously were cultured in DMEM containing 5% FCS [55] . Human melanocyte lines (HEMa-LP, HEMa-DP and HEMn-LP) were purchased from Banksia Scientific (Bulimba, QLD, Australia) and cultured as previously described [56] . Human fresh melanoma isolates were prepared from fresh surgical specimens according to published methods [57] . TMAs were constructed from formalin-fixed paraffin-embedded melanocytic tumour tissues retrieved from the Department of Tissue Pathology and Diagnostic Oncology at the Royal Prince Alfred Hospital, Australia ( Supplementary Table S1 ). Studies using human tissues were approved by the Human Research Ethics Committees of the University of Newcastle and Royal Prince Alfred Hospital, Australia. Melanoma-inducible PIB5PA expression system A lentivirus-based inducible gene expression system described previously was used to express PIB5PA in response to 4-OHT, conditionally in melanoma cells [38] . Briefly, the system involves coinfection of two lentiviral particles: one encoding the inducible transcriptional activator Gal4 1-147 ER T2 VP16 (GEV16) cloned into pFU-GEV16-PGK-Hygro containing a hygromycin-B resistance gene, and another, the PIB5PA complementary DNA cloned into pF-5xUAS-SV40-puro containing a puromycin resistance gene. Dual antibiotic selection was applied, deriving a cell population carrying both GEV16 and PIB5PA. Melanoma xenograft mouse model ME1007.PIB5PA and Mel-FH.PIB5PA cells with or without cointroduced with myr-Akt constructs were treated with vehicle control (dimethyl sulphoxide) or 4-OHT (10 nM) for 36 h. Cells (1 × 10 7 ) were then injected subcutaneously into each flank of male athymic nude mice (Model Animal Research Centre of Nanjing University, China). Two days later, mice were treated with vehicle control (dimethyl sulphoxide) or 4-OHT (10 nM g −1 ) by intraperitoneal injection every 3 days. Mice were killed and tumours weighed at 36 days after tumour cell transplantation. Studies on animals were approved by the Animal Research Ethics Committee of University of Science and Technology of China. Immunohistochemistry Immunohistochemical staining was performed on a Dako autostainer (Dako, Denmark). Antigen retrieval was performed in a pressure cooker for 30 s at 125 °C. Antibody detection was performed using the Dako Envision HRP Detection system/DAB as per the manufacturer’s instructions. Slides were counterstained with Azure B to differentiate the melanin from the brown DAB immunolabelling and haematoxylin. Quantification of immunostained cells was performed as described previously [58] . Immunoblotting Immunoblotting was carried out as described previously [8] , [56] . The intensity of the bands was quantified using the NIH Image J. BrdU proliferation assays BrdU cell proliferation assays were carried out using an assay kit (Cell Signalling) as per the manufacturer’s instructions. Briefly, cells seeded at 5 × 10 3 per well in 96-well plates overnight before treatment as desired. BrdU (10 mM) was added and cells were incubated for 4 h before BrdU assays were carried out. Absorbance was read at 450 nm using a Synergy 2 multi-detection microplate reader (BioTek, VT). Apoptosis Quantification of apoptotic cells was carried out by measurement of sub-G1 DNA content using propidium iodide on a flow cytometer as described elsewhere [8] . Clonogenic assays Cells were seeded at 2,000 per well onto six-well culture plates and allowed to grow for 24 h followed by the desired treatment. Cells were then allowed to grow for a further 12 days before fixation with methanol and staining with crystal violet (0.5% solution). Anchorage-independent cell growth Melanocytes (5 × 10 4 ) harbouring scramble, PTEN or/and PIB5PA shRNA were seeded in 0.3% cell agar layer, which was on top of 0.6% base agar layer in 12-well culture plates. Cells were then incubated for a further 30 days at 37 °C and 5% CO 2 . Cell colony formation was then examined under a light microscope. Chromatin immunoprecipitation assays ChIP assays were performed using the anti-HDAC2, HDAC3, Sp1, acetyl-Histone H3 and H4, and ChIP assay kits (Millipore) according to the manufacturer’s instructions. Briefly, cells were cross-linked using 1% formaldehyde. The bound DNA fragments were subjected to PCR reactions using the following primer pairs: INPP5J , 5′-GCA GTA GGA GTG GAG AGG-3′(sense) and 5′-AGG GCC TCA GAG ACA ACT-3′(antisense); beta-actin (control), 5′-AGC CTT CCT TCC TGG GCA TG-3′(sense) and 5′-CCG ATC CAC ACG GAG TAC TTG C-3′(antisense). Plasmid vectors and transfection The pCGN-PIB5PA-HA and pCGN-PIB5PA SKICH -HA constructs were generous gifts from Christina A. Mitchell (Monash University, Victoria, Australia). The pcDNA-myr-HA-Akt construct was purchased from Addgene (Plasmid 9017). The pCMV6-XL5-PTEN construct was purchased from Origene (SC119965). Cells were transfected with 2 μg plasmid as well as the empty vector in Opti-MEM medium (Invitrogen) with Lipofectamine 2000 reagent (Invitrogen) according to the manufacturer’s protocol. Short hairpin RNA Human PIB5PA shRNA kit (TG310438), human PTEN shRNA kit (TG320498), human Akt shRNA kit (TG320629) and scramble shRNA kit (TG300130), in which shRNA constructs are in retroviral GFP vector (pGFP-V-RS), were purchased from Origene, and were used to infect cells according to the manufacturer’s protocol. Quantitative reverse transcription–PCR Quantitative reverse transcription–PCR analysis was performed as described previously [8] . Assay-on-demand for PIB5PA (assay ID: Hs00300155_m1), PTEN (assay ID: Hs02621230_s1), HDAC1 (assay ID: Hs02621185_s1), HDAC2 (assay ID: Hs00231032_m1), HDAC3 (assay ID: Hs00187320_m1) and GAPDH (assay ID: Hs99999905_m1) were used according to the manufacturer’s protocol (Applied Biosystem). Small RNA interference The siRNA constructs for PIB5PA, PTEN, HDAC1, HDAC2 and HDAC3 were obtained as the siGENOME SMARTpool reagents (Dharmacon, Lafayette, CO), the siGENOME SMARTpool PIB5PA (M-009108-01-0010), the siGENOME SMARTpool PTEN (M-003023-02-0010), the siGENOME SMARTpool HDAC1 (M-003493-02-0010), the siGENOME SMARTpool HDAC2 (M-003495-02-0010), the siGENOME SMARTpool HDAC3 (M-003496-02-0010) and the SiConTRol Non-targeting siRNA pool (D-001206-13-20). Transfection of siRNA pools was carried out as described previously [8] . Luciferase reporter assays The −2,016/+114 fragment of the INPP5J promoter was cloned by genomic PCR using human genomic DNA as a template. The fragment was then cloned into promoterless luciferase reporter plasmid pGL3-Basic Luciferase Vector (Promega). Cells were transiently transfected with pGL3-vector or pGL3- INPP5J with or without cotransfection desired constructs. Luciferase activity was measured using a Synergy 2 multi-detection microplate reader (BioTek, VT) and normalized to the protein content. Exon sequencing Genomic DNA was isolated from melanoma cell lines according to manufacturer’s instructions (Promega). Samples were sequenced using INPP5J exon primers, and data were compared with consensus PIB5PA exon sequence. Quantitative PCR analysis of copy number variations Genomic DNA was extracted from melanoma cells and normal melanocytes. DNA was quantified using a NanoDrop spectrophotometer, and quality was assessed by agarose gel electrophoresis. The specific primers used to examine copy number variations of INPP5J were: forward, 5′-CAAATACGATACCAGGTGAGC-3′; reverse, 5′-GGATACGGTCT GTCCAAGC-3′. As a control, the housekeeping HBB was amplified and quantified. The primers for HBB were: forward, 5′-ACACAACTGTGTTCACTAGC-3′; reverse, 5′-CAACTTCATCCACGTTCACC-3′. Statistical analysis Statistical analysis was performed using JMP Statistics Made Visual software. Student’s t -test was used to assess differences in the expression of the proteins between different groups of melanocytic tumours. The Pearson’s correlation coefficient method was used to test for correlations. A P -value less than 0.05 was considered statistically significant. How to cite this article: Ye, Y. et al . PI(4,5)P2 5-phosphatase A regulates PI3K/Akt signalling and has a tumour suppressive role in human melanoma. Nat. Commun. 4:1508 doi: 10.1038/ncomms2489 (2013).